Ancestral repeats have shaped epigenome and genome composition for millions of years inArabidopsis thaliana Little is known about the evolution of repeated sequences over long periods of time. Using two independent approaches, we show that the majority of the repeats found in the Arabidopsis thaliana genome are ancient and likely to derive from the retention of fragments deposited during ancestral bursts that occurred early in the Brassicaceae evolution. We determine that the majority of young repeats are found in pericentromeric domains, while older copies are frequent in the gene-rich regions. Our results further suggest that the DNA methylation of repeats through small RNA-mediated pathways can last over prolonged periods of time. We also illustrate the way repeated sequences are composted by mutations towards genomic dark matter over time, probably driven by the deamination of methylcytosines, which also have an impact on epigenomic landscapes. Overall, we show that the ancient proliferation of repeat families has long-term consequences on A. thaliana biology and genome composition. Eukaryotic genomes commonly comprise variable amounts of repeated and repeat-derived sequences, including transposable elements (TEs), endogenous viruses, simple repeats, ribozymes and multi-copy gene families. Because of their relative high duplication rate as compared with other genomic components, TEs are typically predominant among eukaryotic repeated sequences [1] and thereby largely contribute to haploid genome size variations [2] . Whereas TEs are thought to be important for the generation of genetic diversity among populations in changing environments [3] , [4] , [5] , their proliferation in evolutionary stable species is potentially deleterious, as they can insert within or nearby genes and hence disrupt host functionalities and regulatory elements [6] . Eukaryotes have evolved various strategies that, to some extent, permit to limit the proliferation of the remaining copies [7] . In several eukaryotic groups, it is thought that DNA methylation on cytosine residues allows transcriptional gene silencing (TGS) of TEs [8] . In Arabidopsis , the methylation of repetitive DNA sequences occurs in three different contexts: CG, CHG and CHH (where H stands for A, T or C) [9] , [10] . The targeting of DNA methylation can be mediated by small RNAs (sRNAs) through the RNA-directed DNA methylation (RdDM) [8] , [11] and NERD [12] , [13] (or RDR6-RdDM) pathways. As a side effect, the transcriptional silencing of repeats can potentially affect the expression of neighbouring genes by establishing repressive chromatin contexts and, in some cases, DNA methylation can even spread within flanking host genes [14] . The model plant A. thaliana is a well-established reference for the study of genome evolution, repetitive DNA and epigenetics in plants. However, little is known about the long-term evolution of repeats in plants. In this work, we determine that most repeated sequences in A. thaliana are relatively old. We use this information to show that both young and old repeats are more frequent in the vicinity of genes with low expression levels. We also show that a substantial pool of sRNAs corresponds to old repeats, suggesting that repeat sequence divergence is accompanied by a diversifying population of sRNAs. In corollary, we find significant levels of DNA methylation in the old RdDM-targeted repeats. Our results further propose a possible link between RdDM and G+C content. Finally, we present results illustrating that the repeated sequences may evolve in a bimodal fashion with mutation rates first dominated by the deamination of methylcytosines and then by the basal endogenous rates of transitions and transversions. Divergence and distribution of A. thaliana repeats A critical issue to assess genome evolution is to discriminate between repeats that integrated recently (young repeats) from those that have inserted relatively long ago (old repeats). The evolution of repeat families follows a ‘burst and decay’ model with the proliferation of identical copies that, once transposed, accumulate mutations and deletions randomly and separately from other copies. The generation of consensus sequences from the information contained in multiple copies enables to reconstruct the ancestral sequence of a repeat family. As a result, the divergence between genomic copies and consensus sequences enables to roughly approximate the relative age of the copies. Indeed, the alignment of several close to identical (young) copies generates a closely related consensus sequence, while a consensus derived from the alignment of a set of more divergent (old) copies is more distant to all the copies. Here we have first built consensus sequences from families of repeated segments found in the A. thaliana genome (accession Col-0) and used them to annotate the whole genome with coverage of 28.9 Mb (24.3%). This amount is similar to a recent estimate using the same pipeline [15] . We then measured the identity between repeat copies in the A. thaliana genome and cognate consensus sequences to assign relative copy ages following the simplest substitution model. We found that the vast majority (over 73%) of A. thaliana copies has <85% identity with the respective consensus sequence, and that these together contribute c. 52% of the repeat space. In contrast, we found that only 10.5% of the copies were detected with high identity ( ⩾ 95%) matches ( Fig. 1a ), while these collectively contribute ~26% of the repeat space. The finding of mostly substantially divergent repeat copies in A. thaliana is consistent with relatively limited recent TE activity in this species [16] , [17] and suggests the prevalence of ancient elements. In contrast, previous analyses have reported evidences of recent and massive bursts in the close relative Arabidopsis lyrata that postdate the separation with A. thaliana 5–10 million years ago (mya) [18] , [19] . In strong support to the relevance of the divergence-based approach applied to A. thaliana , the same analysis performed on the A. lyrata genome indeed reveals a neat peak in the frequency of high pairwise identities between copies and consensus sequences ( Fig. 1a ). 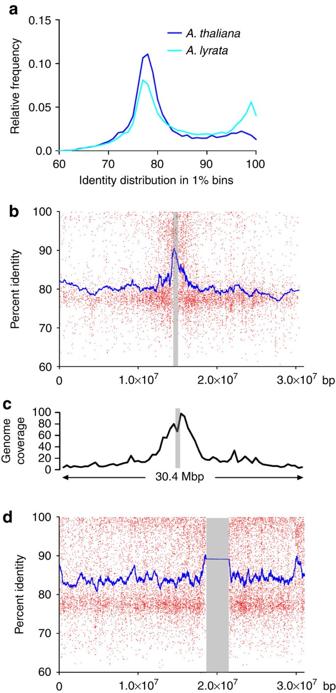Figure 1: Identification and distribution of divergent repeats inA. thaliana. (a) Distribution in 1% bins of the identity values between genomic copies and consensus sequences inA. thalianaandA. lyrata.(b) Plot (red dots) and smoothed curve (blue line) of the identities between genomic copies and consensus sequences alongA. thalianachromosome 1 (30.4 Mbp). Grey shading indicates the centromere. (c) Repeat coverage (per cent per 500-kb bins) along theA. thalianachromosome 1 drawn to scale withb. Grey shading indicates the centromere. (d) Plot (red dots) and smoothed curve (blue line) of the identities between genomic copies and consensus sequences alongA. lyratachromosome 1. Grey shading indicates that centromeres are not assembled for this species. Figure 1: Identification and distribution of divergent repeats in A. thaliana . ( a ) Distribution in 1% bins of the identity values between genomic copies and consensus sequences in A. thaliana and A. lyrata. ( b ) Plot (red dots) and smoothed curve (blue line) of the identities between genomic copies and consensus sequences along A. thaliana chromosome 1 (30.4 Mbp). Grey shading indicates the centromere. ( c ) Repeat coverage (per cent per 500-kb bins) along the A. thaliana chromosome 1 drawn to scale with b . Grey shading indicates the centromere. ( d ) Plot (red dots) and smoothed curve (blue line) of the identities between genomic copies and consensus sequences along A. lyrata chromosome 1. Grey shading indicates that centromeres are not assembled for this species. Full size image We next addressed the distribution of the identity values along the A. thaliana chromosomes and we found that the vast majority of high identity matches are located within pericentromeric regions ( Fig. 1b and Supplementary Figs 1–4 ). This landscape correlates positively with the density of repeated sequences (Fig. 1c and, Supplementary Figs 1–4 ). Pericentromeric regions also appear to contain a vast amount of older copies. Instead, the repeat-poor regions appear to be populated almost exclusively by old copies ( Fig. 1b,c ). In contrast, we observe a distinct distribution in A. lyrata for which young repeats are frequent all along the chromosomes ( Fig. 1d ). We thus find differential repeat divergence in gene-dense (chromosome arms) versus gene-poor (pericentromeric) regions. Although these results suggest the presence of essentially old repeats in gene-rich regions of the A. thaliana genome, we cannot rule out that apparent enhanced divergence could be the result of an accelerated evolutionary pace of repeats in gene-dense regions. A legacy from ancestral bursts After separation from a common ancestor, repeat families have different destinies in different plant genomes. For example, a specific repeat family can multiply again in one species and not in another one. The burst of an autonomous repeat family is a highly selective process: only the copies that have accumulated limited mutational drift are functional and are capable to burst [1] . Such a selective burst allows the multiplication of the best conserved copies, that is, the ones that are closest to the ancestral sequence. Therefore, the TE families that maintain active in some genome should longer preserve the ancestral sequence as compared with a decaying pool of relatives in another genome ( Supplementary Fig. 5A ). As a consequence, a repeat copy from one species is most likely to be relatively old if it is most similar to a consensus sequence established from a foreign species. We tried to take advantage of this theory to confirm the relative age distributions documented above ( Fig. 1 ). The genome of several A. thaliana relatives that diverged ~5–40 mya [20] , [21] have been sequenced: A. lyrata , Capsella rubella , Arabis alpina , Brassica rapa , Thellungiella salsuginea (formerly Thellungiella halophila ) and Schrenkiella parvulum (formerly Thellungiella parvula ) [18] , [22] , [23] , [24] , [25] , [26] ( Supplementary Fig. 5B ). The genomes from four other A. thaliana ecotypes have been assembled (Ler-1, Kro-0, Bur-0 and C24) [27] as well. For all these genomes, we have generated a library of consensus repeat sequences that we appended to the Col-0 library to compile a ‘ Brassicaceae ’ library that was used to annotate the Col-0 genome. The Brassicaceae annotations cover over 46 Mb of the A. thaliana genome to which coding DNA sequences (CDS) contribute nearly 20% (9 Mb). This effect was anticipated, as the Brassicaceae library likely comprises the cumulative sets of species-specific repeated host genes. Nevertheless, the Brassicaceae annotations appear to achieve highly sensitive detection of repeated and repeat-derived sequences ( Supplementary Fig. 5C , see Methods) and we further focus on the subset that does not overlap with CDS (~31.8 Mb). Importantly, although in theory a single copy in the genome can be detected by several similar consensus sequences in a library, the annotation programme applies a ‘consensus with best score wins’ rule. Thus, although the construction of the Brassicaceae library inherently supposes the collection of related sequences from different species, each annotation in the A. thaliana genome will be attributed to the closest consensus. In such a competitive context, we found that most of the copies that were detected previously ( Fig. 1a ) with <~85% identity have now been detected with better scores by sequences fetched from other Brassicaceae species ( Fig. 2a ). This result strongly supports the relevance and the power of such a pan-species, competitive approach for repeat annotation. 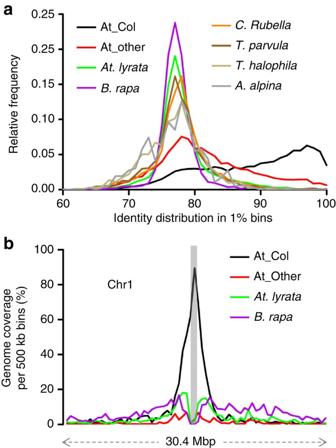Figure 2: Ancestral repeats in theA. thalianagenome. (a) We performed a competitive annotation of theA. thalianagenome with theBrassicaceaelibrary: each copy being detected by the most similar consensus sequence (best score) and resulting inA. thalianacopies being attributed to differentBrassicaceaespecies. For each species, we plot the distribution of identity values between genomic copies and consensus sequences in 1% bins (‘At_other’ represents the pool of Ler-1, Kro-0, Bur-0 and C24 accessions). (b) Distribution along the Col-0 chromosomes of the contributions of the annotations attributed to consensus sequences from different species and ecotypes (‘At_other’ represents the pool of Ler-1, Kro-0, Bur-0 and C24). Grey shading indicates the centromere. Figure 2: Ancestral repeats in the A. thaliana genome. ( a ) We performed a competitive annotation of the A. thaliana genome with the Brassicaceae library: each copy being detected by the most similar consensus sequence (best score) and resulting in A. thaliana copies being attributed to different Brassicaceae species. For each species, we plot the distribution of identity values between genomic copies and consensus sequences in 1% bins (‘At_other’ represents the pool of Ler-1, Kro-0, Bur-0 and C24 accessions). ( b ) Distribution along the Col-0 chromosomes of the contributions of the annotations attributed to consensus sequences from different species and ecotypes (‘At_other’ represents the pool of Ler-1, Kro-0, Bur-0 and C24). Grey shading indicates the centromere. Full size image When measuring the coverage of the non-CDS Brassicaceae annotations attributed to consensus sequences from each species, we found that although Col-0 contributes the largest part (36.8%), A. lyrata and B. rapa contribute as much as 17.5 and 25.8%, respectively, with modest (below 6.5%) contributions from other species and the pool of non-Col-0 A. thaliana ecotypes ( Supplementary Fig. 6 ). In other words, the majority of the non-CDS Brassicaceae annotations in the A. thaliana genome correspond to regions that are better detected by consensus sequences constructed from other species. Nevertheless, the majority (76%) of these regions have been detected by Col-0 consensus when not competing with sequences from other species. The fact that most A. thaliana copies can be detected more accurately by consensus sequences built in foreign species is most parsimoniously explainable by shared ancestry, which indicates the long decay of these copies in A. thaliana . We further examined the distribution of the non-CDS Brassicaceae annotations along the A. thaliana chromosomes, with focus on the occurrences attributed to consensus from A. lyrata , B. rapa and non-Col-0 accessions ( Fig. 2b and Supplementary Fig. 7 ). Interestingly, we found that the annotations that are attributed to consensus sequences from A. thaliana are almost restricted to pericentromeric regions (including the knob located on the short arm of chromosome 4 (ref. 28 )). Instead, those attributed to consensus sequences from B. rapa are skewed towards ‘outer’ pericentromeric regions and chromosome arms ( Fig. 2b and Supplementary Fig. 7 ). In striking contrast, after annotating the A. lyrata genome with the Brassicaceae library we found that consistent with recent repeat proliferation in this genome [18] , most (64%) of the non-CDS annotations (70 Mb) are attributed to consensus sequences from A. lyrata ( Supplementary Fig. 8 ) and that these copies are most frequent all along the A. lyrata chromosomes ( Supplementary Fig. 9 ). The present analysis therefore provides independent evidences supporting the ancient origin of the A. thaliana repeats as well as the chromosome-level distribution of old versus young copies in this species. The ‘old’ sRNA pool The results presented above provide an opportunity to compare the populations of A. thaliana sRNAs corresponding to young versus old copies in order to gain insights on the adaptation of repeat regulatory pathways over time. Here we arbitrarily discriminate young and old repeats as those showing respectively more or less than 85% identity with the cognate consensus sequence following genome annotation with the Col-0 library alone (see the first Results section, Fig. 1a ). The RdDM pathway is known to perform de novo methylation on repeated sequences through targeting by 24-nucleotide (nt) sRNAs [8] , [11] . To investigate to what extent young versus old repeats would be affected by RdDM, we compared their positions to those of 24 nt features from a map of sRNAs in A. thaliana [10] . We first observed that although virtually all (89%) young repeats overlap with the 24-nt sRNA map (hereafter referred to as 24-nt sRNA+ repeats), 50% of the old repeats do ( Fig. 3a ). Consistent with the distribution of gene-dense versus gene-poor regions in A. thaliana , we notice that ancient 24-nt sRNA+ repeats are located closer to genes than young 24-nt sRNA+ copies ( Supplementary Fig. 10 , Mann–Whitney U (MWU) P -value<0.0001). We also found that ancient 24-nt sRNA− copies are located closer to genes than young 24-nt sRNA− copies ( Supplementary Fig. 10 , MWU P -value<0.0001). 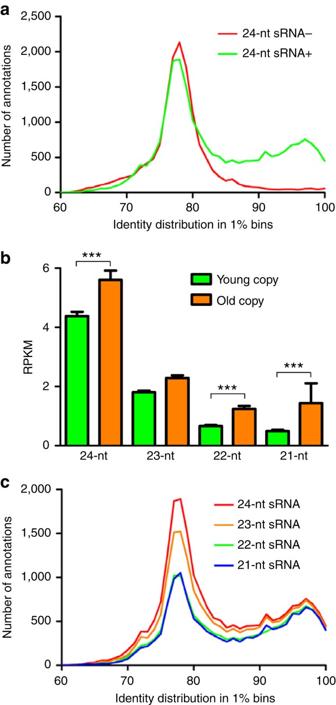Figure 3: Occurrence of sRNAs in old repeats. (a) Distribution in 1% bins of the identity values betweenA. thalianagenomic copies and consensus sequences following whether copies overlap at least one 24-nt sRNA (24-nt sRNA+) or not (24-nt sRNA−). (b) Read density for all sRNA classes addressed in young versus old copies that overlap with at least one read of the respective class. Copy numbers are as follows: N(24-nt sRNA+ young copies)=8,342; N(24-nt sRNA+ old copies)=12,841; N(23-nt sRNA+ young copies)=7,906; N(23-nt sRNA+ old copies)=10,526; N(22-nt sRNA+ young copies)=6,909; N(22-nt sRNA+ old copies)=7,252; N(21-nt sRNA+ young copies)=6,694; N(21-nt sRNA+ old copies)=6,842. Error bars are defined as s.e.m. ***Statistically supported differences (MWUP-value<0.0001). (c) Distribution in 1% bins of the identity values betweenA. thalianagenomic copies and consensus sequences for each class of sRNA addressed. Figure 3: Occurrence of sRNAs in old repeats. ( a ) Distribution in 1% bins of the identity values between A. thaliana genomic copies and consensus sequences following whether copies overlap at least one 24-nt sRNA (24-nt sRNA+) or not (24-nt sRNA−). ( b ) Read density for all sRNA classes addressed in young versus old copies that overlap with at least one read of the respective class. Copy numbers are as follows: N(24-nt sRNA+ young copies)=8,342; N(24-nt sRNA+ old copies)=12,841; N(23-nt sRNA+ young copies)=7,906; N(23-nt sRNA+ old copies)=10,526; N(22-nt sRNA+ young copies)=6,909; N(22-nt sRNA+ old copies)=7,252; N(21-nt sRNA+ young copies)=6,694; N(21-nt sRNA+ old copies)=6,842. Error bars are defined as s.e.m. ***Statistically supported differences (MWU P -value<0.0001). ( c ) Distribution in 1% bins of the identity values between A. thaliana genomic copies and consensus sequences for each class of sRNA addressed. Full size image The fact that one repeat copy overlaps with a single 24-nt sRNA position is not necessarily biologically relevant so we compared the density of 24-nt sRNA features over young versus old repeats. Unexpectedly, we found that, among the 24-nt sRNA+ copies, the density of 24-nt reads (number of reads per kilo base per million) is significantly higher for old copies as compared with the young ones ( Fig. 3b , MWU P -value<0.0001). This is consistent with the previously reported higher density of 24-nt sRNAs that match repeats located along chromosome arms as compared with those that match repeats in pericentromeric regions [14] . We addressed whether the differences observed could be biased or smoothened by multiply mapping 24-nt sRNA that would target both young and old copies. We found that only 8% of the different sRNA molecules cross-match both repeat types, thus introducing only a limited bias in this comparison. DNA methylation can also be guided by 21- and 22-nt sRNA species in the non-canonical RdDM pathway referred to as ‘NERD’ or ‘RDR6-RdDM’ pathway [12] , [13] . In addition, 21- and 22-nt sRNA species could contribute to repeat post-TGS [29] . We found that although the majority (79%) of young repeats overlaps the positions of 21-nt sRNAs, only a subset of older repeats does (29%) ( Fig. 3c ). Nonetheless, among the copies that overlap the position of at least one 21-nt sRNA, we observed that on average the read density is significantly higher for old repeats as compared with young ones ( Fig. 3b , MWU P -value<0.0001). A similar significant distinction holds for 22-nt sRNAs, whereas it is not statistically supported for 23-nt sRNAs. siRNA-directed DNA methylation occurs in all sequence contexts (CG, CHG and CHH) and siRNAs target ca . 30% of all mC in A. thaliana [9] , [10] . Consistently, although crossing sRNA data derived from inflorescences [10] and bisulphite sequencing data derived from root tissues [30] , we found conspicuous evidence that the level of CG methylation in old 24-nt sRNA+ repeats is significantly higher than the one observed in old copies that are not 24-nt sRNA targets ( Supplementary Fig. 11A , MWU P -value<0.0001). A similar difference was observed in young 24-nt sRNA+ versus young 24-nt sRNA− copies and we found that these differences also apply to CHG and CHH methylation levels in both young and old repeat sets ( Supplementary Fig. 11B,C , MWU P -values<0.0001). Overall, our results suggest that repeat copies of different ages are significantly methylated in all sequence contexts provided that they are targeted by 24-nt sRNAs. Gene expression levels analysis We addressed the expression levels of genes that are associated to repeated elements. We first observed that on average younger repeats are located further from genes as compared with older ones and this trend holds using the two dating proxies described above ( Supplementary Fig. 12 ). Again, this is in line with the fact that young insertions are mostly found in the gene-poor pericentromeric regions. We next assessed whether genes associated with young versus old repeats have different expression levels. On average, we found that genes with flanking repeat (<500 bp to the upstream or downstream closest repeat) are expressed at lower levels as compared with repeat-free genes ( Fig. 4a , MWU P -value<0.0001). Furthermore, genes carrying a repeat are expressed at even lower levels, on average (MWU P -value (repeat within/repeat-free)<0.0001, MWU P -value (repeat within/flanking repeat)<0.0001). Similar results were reported previously [31] , [32] . Unexpectedly though, we found that genes with old flanking repeat are expressed at similarly low levels than those with young flanking repeat ( Fig. 4b , MWU P -value=1). Likewise, the overall expression level of genes with young repeat within is not significantly different from the one of genes with old repeat within ( Fig. 4b , MWU P -value=0.026). 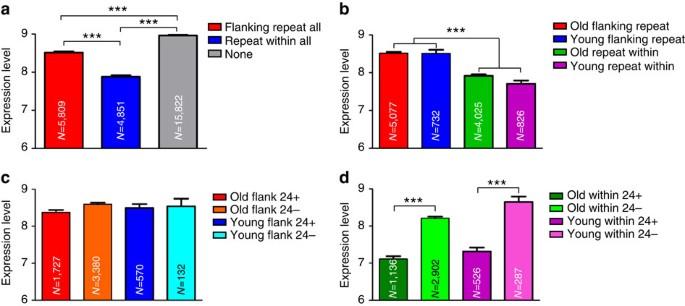Figure 4: Gene expression analysis. (a) Expression levels of theA. thalianagenes with respect to the presence and location of repeats. ***Statistically supported differences (MWUP-value<0.0001). (b) Expression levels of theA. thalianagenes with respect to the presence, location and age of repeats. ***Any of the two sets of gene with flanking repeat is significantly different (MWUP-value<0.0001) from any of the two sets of genes with repeat within. (c) Expression levels of theA. thalianagenes with flanking repeats with respect to the age of repeats and overlap with 24-nt sRNA. (d) Expression levels of theA. thalianagenes carrying repeats with respect to the age of repeats and overlap with 24-nt sRNA. ***Statistically supported differences (MWUP-value<0.0001). For all panels, error bars are defined as s.e.m. Figure 4: Gene expression analysis. ( a ) Expression levels of the A. thaliana genes with respect to the presence and location of repeats. ***Statistically supported differences (MWU P -value<0.0001). ( b ) Expression levels of the A. thaliana genes with respect to the presence, location and age of repeats. ***Any of the two sets of gene with flanking repeat is significantly different (MWU P -value<0.0001) from any of the two sets of genes with repeat within. ( c ) Expression levels of the A. thaliana genes with flanking repeats with respect to the age of repeats and overlap with 24-nt sRNA. ( d ) Expression levels of the A. thaliana genes carrying repeats with respect to the age of repeats and overlap with 24-nt sRNA. ***Statistically supported differences (MWU P -value<0.0001). For all panels, error bars are defined as s.e.m. Full size image We then compared the expression levels of genes that are flanked by young and old repeats following whether they overlap with the 24-nt sRNA map or not. About a third of the old gene-flanking repeats overlap with 24-nt sRNA map, while ~80% of the young gene-flanking repeats do. Nevertheless, we found no statistically supported difference in the transcript levels of genes flanked by old or young repeats whether these are 24-nt sRNA+ or not ( Fig. 4c ). This situation is strikingly different for genes that carry a repeat as their expression levels are overall significantly lower when the repeat overlaps the 24-nt sRNA map, regardless of whether it is old or young ( Fig. 4d ). Two hypotheses could explain the overall correlation between low gene expression levels and the presence of repeats: (i) repeated elements cause low gene expression, (ii) repeated elements are more frequent in the vicinity of low expressed genes; (i) and (ii) not being mutually exclusive. We investigated whether we could detect a causal relationship between the presence of repeated elements and low gene expression levels. In this scope, we first compared the expression levels in the A. thaliana accession Col-0 with those observed for orthologous genes in the accessions C24 and Bur-0, discriminating for the presence/absence of flanking repeats. We found that the differences in gene expression levels between the Col-0 and Bur-0 accessions are not significantly different for the pairs of orthologues that are repeat-free in both accessions and for those that are repeat-proximal in Col-0 and repeat-free in Bur-0 ( Supplementary Fig. 13A , MWU P value=0.16). Likewise, no significant differences were observed when comparing the expression levels of repeat-proximal genes in Col-0 and repeat-free orthologues in C24 ( Supplementary Fig. 13B , MWU P -value=0.42). We also compared the expression levels of orthologous genes that carry a repeat in Col-0 but not in the Bur-0 or C24 accessions. Again, we found that the differences in expression levels between accessions are similar to those observed with the pairs of invariably repeat-free genes (MWU P -value (Col-0 versus Bur-0)=0.56, P -value (Col-0 versus C24)=0.49). Together, these results advocate that hypothesis (ii) proposes the most common explanation for the correlation between repeat presence and low gene expression levels in A. thaliana . The origin and fate of repeats TEs and other repeated and repeat-derived sequences have a general evolutionary tendency towards the suppression of cytosines (C) and guanines (G) that is interpreted as resulting over time from the action of cytosine methylation [33] . Indeed, although cytosine and 5-methylcytosine undergo comparable rates of spontaneous hydrolytic deamination that respectively produce uridine and thymine, the mismatch repair of C→T transitions is less efficient than that of C→U transitions [34] , [35] . Therefore, as in many eukaryotic lineages (including plants) DNA methylation is preponderant in repeated sequences [36] , these have relatively low G+C contents as compared with host genes in various species [37] . Accordingly, we measured 39% G+C in the library of A. thaliana consensus repeats as compared with 44% in CDS. Furthermore, we observe that the overall G+C content is significantly lower (30.50%) in old versus young (37.65%) repeated and repeat-derived sequences. This trend also appears clearly at the whole genome level. Considering the heterogeneous distribution of young and old repeats along the A. thaliana chromosomes, we would expect a correlated distribution of the G+C content. When calculating the G+C content of the concatenated repeat annotations, we obtained profiles that are highly suggestive of significantly lower G+C content in the chromosome arms as compared with pericentromeric regions ( Fig. 5a and Supplementary Fig. 14A ). In contrast, the G+C content of the concatenated CDS appears remarkably stable along the chromosomes ( Supplementary Fig. 14B ). 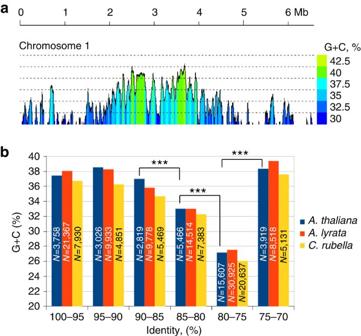Figure 5: Composition of aging repeats. (a) Plot showing the G+C content along the concatenated repeat copies detected on chromosome 1 using the Col-0 library. Gaps indicate values below 30%. (b) Histogram showing average G+C content in the copies distributed in bins of 5% identity with respective consensus sequence. ***Statistically supported differences (MWUP-value<0.0001). Statistical tests were run forA. thalianaonly. Figure 5: Composition of aging repeats. ( a ) Plot showing the G+C content along the concatenated repeat copies detected on chromosome 1 using the Col-0 library. Gaps indicate values below 30%. ( b ) Histogram showing average G+C content in the copies distributed in bins of 5% identity with respective consensus sequence. ***Statistically supported differences (MWU P -value<0.0001). Statistical tests were run for A. thaliana only. Full size image Over time, mC deamination leads to the pauperization of targets of DNA methylation and thus the contribution of deamination-driven mutation decreases as compared with the steady, basal rate of transitions and transversions in A. thaliana . Therefore, we hypothesize that after a significant amount of time, the number of mC reduces to a point that deamination becomes a minor/null force over the whole mutations occurring. At this stage the G+C content of such old sequences may converge back to the mean by following the basal mutational rates in A. thaliana . Remarkably, we observed such an effect when measuring the GC content in bins from a gradient of values of similarity to the consensus. Indeed, although moderately divergent sequences show low G+C content as compared with very young repeats, we found that extensively divergent sequences show a G+C content that is higher than found in young repeats ( Fig. 5b ). Remarkably, we observe a very similar trend when performing the same analysis with the close relatives A. lyrata and C. rubella ( Fig. 5b ). Such a profile could also be due to variations in the initial G+C content of the copies that predominantly integrated at different periods. We have therefore investigated whether the A. thaliana genome contains traces of waves of integration of different repeat families over time. Interestingly, we noticed that the majority of old repeats correspond to putative remnants of Helitron TEs ( Fig. 6a ). Incidentally, this wave overlaps substantially with the overall drop in G+C content detected within old repeats ( Fig. 5b ) and we found that on average, Helitrons are A+T-rich as compared with other classes of repeated sequences, suggesting that such a massive, ancestral burst could significantly contribute to the overall low G+C content observed in old repeats ( Fig. 6b ). Nevertheless, the contribution of specific repeat families and the effect of mutations on the variation of the overall G+C content are not mutually exclusive. We have therefore measured the variation of G+C content of specific repeat families over time and found that several major TE families show a bimodal trend as for the whole repeat pool, although to lesser ranges of variations (MWU P -value [G+C content in 100–95% identity bin/G+C content in 85–80% identity bin]<0.0001 and MWU P -value [G+C content in 85–80% identity bin/G+C content in 75–70% identity bin]<0.0001 for each repeat shown in Fig. 6b ). 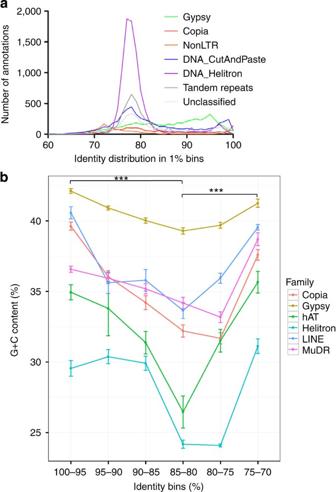Figure 6: G+C content in repeats over time. (a) Distribution in 1% bins of the identity values betweenA. thalianagenomic copies and consensus sequences for different classes of repeats. (b) G+C content in copies from different repeat families distributed in bins of 5% identity with respective consensus sequence. Error bars are defined as s.e.m. ***Statistically supported differences (MWUP-value<0.0001) for all repeat families. Figure 6: G+C content in repeats over time. ( a ) Distribution in 1% bins of the identity values between A. thaliana genomic copies and consensus sequences for different classes of repeats. ( b ) G+C content in copies from different repeat families distributed in bins of 5% identity with respective consensus sequence. Error bars are defined as s.e.m. ***Statistically supported differences (MWU P -value<0.0001) for all repeat families. Full size image Following this model, deamination is expected to remain a significant mutational force for the 50% of old repeats that are 24-nt sRNA+ and hence supposedly targeted by the RdDM pathway. We addressed whether there is a significant difference in G+C content of the old repeats depending on whether they are targeted by 24-nt sRNAs or not. In support of a correlation between G+C content and de novo cytosine methylation, we found that on average G+C content in old 24-nt sRNA+ repeats is significantly higher than in old 24-nt sRNA− repeats (MWU P -value<0.0001), while it is similar in young 24-nt sRNA+ versus young 24-nt sRNA− copies ( Supplementary Fig. 15 ). This observation further supports the bimodal mutational bias followed by aging repeat copies. We speculate that after a prolonged period of time, G+C content reaches a critically lower threshold that let copies shift beyond the RdDM ‘radar’. Once deserted by the RdDM machinery, old copies could undergo increasing GC content following the basal mutational rate. In this work, we have determined that most of the A. thaliana repeats are ancient. These results are in strike contrast with those from a previous study [38] , which proposed that most TE copies in A. thaliana are young. However, the authors of this work had used two different proxies to infer rough copy dating. First, population frequency, arguing that fixed TE insertions should be older than polymorphic insertions. However, considering the apparent ongoing A. thaliana genome reduction we estimate that although polymorphic insertions may reflect new insertions, they may also reflect the loss of older insertions and thus may not reliably help to estimate copy age. Second, Hollister et al . [38] considered insertions that are unique to A. thaliana as relatively young as compared with insertions that are shared between A. thaliana and A. lyrata . In the light of our work, this method appears to be somewhat erroneous as both species are likely to retain highly variable fractions of the ancestral copies. Indeed, the virtually opposite TE dynamic in the two species since their separation suggests highly unequal turnover and conservation rate of ancient repeats such that the non-conservation of insertions in the two species is not expected to reflect their age. Here we do not employ the popular dating approach that is widely applied in plants consisting in estimating insertion date based on the divergence between pairs of long-terminal repeats (LTRs) from LTR elements, being identical on insertion and then accumulating mutations. There are several reasons to this. First this method is calibrated on substitution rates measured in a few host genes and ‘anonymous’ intergenic regions in rice [39] . It therefore seems hardly applicable when dealing with deamination-driven mutational biases for different repeat families in different species. Second, this method can only assess the divergence of LTR elements, although we do not expect equivalent dynamics for all repeat families at different times during evolution. Third, this method inherently applies only to (near) full-length elements as LTRs need to be present at both extremities of an element, thereby discarding the vast majority of the copies that have undergone deletions and insertions through time. Therefore, measuring the divergence of any copy with its cognate consensus sequence appears to be a more comprehensive approach in terms of ranges of ages and families assessed, as commonly applied with mammalian genomes [40] , [41] , [42] , [43] , [44] where more complex strategies have confirmed the relative ages of repeated elements obtained from divergence-based approaches [45] . In this work, we chose not to apply any specific substitution model to perform a neutral analysis as we cannot anticipate the different molecular clocks applying over time and between original repeats. We can nevertheless make some estimates of the age of repeat copies in A. thaliana . Ossowski et al . [46] have recently calculated an average rate of 7 × 10 −9 substitution per site per generation in A. thaliana on the basis of mutations accumulated in the whole genome after 30 generations (most of which being found in TEs). Applying this number to evolutionary distances obtained using the Kimura two-parameter model [47] , we found that most A. thaliana repeats are over 30 million years old ( Supplementary Fig. 16 ). Ma et al . [48] proposed an almost twice higher rate (1.3 × 10 −8 substitution per site per generation) for neutral sequences in rice which, when applied to A. thaliana repeats, suggests that most copies are over 15 million years old ( Supplementary Fig. 16 ). Our Brassicaceae library allows determining that over 50% of the non-CDS A. thaliana repeats (in terms of coverage) is detected with better scores by consensus sequences from other Brassicaceae species ( Fig. 2 ). This first suggests that the repeat families involved were present in an ancestral genome that predates the A. thaliana – A. lyrata separation. Furthermore, ~35% of the non-CDS A. thaliana annotations are attributed to consensus identified in genomes from the Arabis , Brassica and Eutrema groups, suggesting that related repeats were present 25–40 mya [20] , [21] in a Brassicaceae paleogenome ( Supplementary Fig. 5B ). The consensus from B. rapa outcompete those from other foreign Brassicaceae for repeat detection in A. thaliana ( Supplementary Fig. 6 ). This could be related to the triplication of the B. rapa genome c . 10–15 mya [49] , [50] that may have generated a number of repeat-tolerant regions as reserves for a variety of repeats. Along the A. thaliana chromosome arms, the contribution of the annotations attributed to B. rapa exceeds the ones from less divergent species, again supporting the fixation of ancient repeats in gene-rich domains ( Fig. 2b and Supplementary Fig. 7 ). Our competitive approach thereby exemplifies the variable preservation of repeat families among species deriving from a common ancestor and fits the apparent ongoing genome reduction and the limited recent TE activity in A. thaliana [16] , [17] , [51] . As described recently, we found that the transcriptional levels of repeat-free genes are on average higher than that of repeat-flanking genes and to a greater extent than that of repeat-containing genes [31] , [32] . However, comparison of gene expression levels in Col-0 and two other accessions (Bur-0 and C24) failed to identify a causal relationship between repeat presence and low expression levels. This proposes that overall the selective pressure against repeated elements is negatively correlated with gene expression levels and that the repeats still present in the A. thaliana genome have modest impacts on gene expression. The discrepancy with a recent publication [32] may be attributable in the first place to the different methods used to annotate (or call) genes and repeats in the Bur-0 and C24 accessions. Among the bulk of genes assessed here, the average trend is likely to hide peculiar cases of genes, which expression is indeed regulated by the presence of repeats, including cases in which this process is adaptive and conserved in different accessions such as for the fwa gene [52] . After the recent description of the sequence of events leading to de novo silencing of the Evadé retrotransposon [29] , we describe here that sRNA-mediated DNA methylation of repeated sequences appears to last over long evolutionary periods. If the RdDM-driven taming of some repeat copies was to remain substantial over time, sequence divergence and decreasing cytosine targets due to deamination-driven mutations [46] postulates the need for an increasing diversity of 24-nt sRNA over time. Nonetheless, although virtually all young repeats overlap the 24-nt sRNA map studied here, the proportion of the old copies that do not overlap this map comes to roughly 50%, suggesting that the proportion of copies undergoing RdDM decreases with time. Besides 24-nt sRNA, we found a similar general scheme for 21- and 22-nt sRNA classes, suggesting that old repeats may also be the targets of post TGS and/or the recently described RDR6-RdDM pathway [12] , [13] , [29] . Silencing old repeats is unexpected as they are probably severely compromised by millions of years of mutational drift and deletions so that the bulk of these sequences are most likely harmless. Indeed, the analysis of A. thaliana mutants for enzymes of the methylation pathway show that only a limited subset of TEs is actually capable to proliferate [53] , [54] . Hypothetically, as representing a highly diversified pool of sRNA sources, old repeats could provide a safeguard reservoir that could potentially help fighting against emerging new species of younger relatives. Data sets Genome sequences were obtained from the following sources: A. thaliana ecotype Col-0 (TAIR10 release) ( http://www.phytozome.com/arabidopsis.php ); A. thaliana ecotypes Ler-1, Kro-0, Bur-0, and C24 ( http://www.1001genomes.org/ ); A. lyrata (v1.0, http://www.phytozome.com/alyrata.php ); C. rubella (initial release, http://www.phytozome.com/capsella.php ); A. alpina ( https://urgi.versailles.inra.fr/download/AaGenomeV4.tar.gz ); T. parvula (v2.0, http://thellungiella.org/data/ ); T. halophila (initial release, http://www.phytozome.com/thellungiella.php ); B. rapa (v1.2, http://www.phytozome.com/napacabbage.php ). The sRNA map used in this work corresponds to data set GSM277608 from the Gene Expression Omnibus (GEO) database ( http://www.ncbi.nlm.nih.gov/geo/ ) with lift up to TAIR10 assembly. The occurrences of multiply mapping reads were distributed evenly among genomic copies. Normalized expression data for the Col-0, Bur-0 and C24 ecotypes were kindly provided by Xi Wang and Detlef Weigel [32] , and derived from the raw data available in GEO data set GSE24669. Both the sRNA and expression data sets derive from inflorescences of plants grown at 23 °C with 16 h light period. The DNA methylation data corresponds to the average values in 50 bp windows from GEO GSM1014124. This data set derives from 3-week-old root tissues of Col-0 plants grown under a 16-h light period. The reference gene data set corresponds to TAIR10 ( ftp://ftp.arabidopsis.org/Maps/gbrowse_data/TAIR10/ ). This data set derives inflorescences of plants grown at 23 °C with 16 h light period. TE genes and pseudogenes were filtered from this data set. Host gene expression levels were computed from published data using tiling 1.0R arrays for biological triplicates from Col-0 inflorescences [32] . Genome annotation For all the Brassicaceae addressed, including the A. thaliana Col-0, Bur-0 and C24 accessions, we have used the TEdenovo pipeline from the REPET package (v2.0) with default parameters [15] . Consensus sequences derived from LTR Harvest predictions were retained only when they presented pfam domains typical of LTR retrotransposons. Classification of the consensus sequences was performed using the REPET utility by looking for characteristic structural features and similarities to known TEs from Repbase (17.01) [55] , and by scanning against the Pfam library (26.0) [56] with HMMER3 (ref. 57 ). Genome annotation was done with the TEannot pipeline [58] from REPET with default settings. Values of identity between input consensus sequences and annotated copies were collected directly from the output of the TEannot pipeline. To assess the sensitivity of the A. thaliana annotations using the Brassicaceae library, we have compared them with a variety of independent, repeat-rich data sets, including annotations using the RepeatModeler (Smit and Hubley, 2008–2010, RepeatModeler Open-1.0. http://www.repeatmasker.org ), RepeatScout [59] and tallymer [60] programmes, as well as the map of 24-nt sRNA and annotations obtained using the reference A. thaliana repeats from Repbase [55] and a set of manually curated consensus sequences [61] . We measured the coverage off all these data sets by the Brassicaceae annotations ( Supplementary Fig. 5C ). When running the TEannot pipeline on the Bur-0 and C24 accessions, accession-specific consensus sequences were pooled to the ones identified in Col-0 to build respective input libraries with limited bias due to the poor assembly of repeated elements in the genome assemblies of the Bur-0 and C24 accessions [27] that a priori does not allow comprehensive initial detection of repeats used for the construction of consensus sequences. Data processing and filtering Only the annotations measuring at least 100 bp were kept for calculation of similarity with consensus, distance to genes, sRNA density and G+C content. Although the TEannot pipeline performs a ‘long join’ procedure to try to connect fragments that may have been interrupted after insertion, our analyses were run directly on each fragment. Coverages, differences, distances and overlaps between data sets were computed using the S-MART suite [62] . To estimate ages of insertions, each copy was re-aligned to its cognate consensus sequence using ‘Needle’ sequence aligner and evolutionary distances were calculated with ‘Distmat’ using Kimura two-parameter model, both programmes being from the Emboss package [63] . We identified the positions of Col-0 ortholgues in the Bur-0 and C24 accessions by comparing the Col-0 genes to the Bur-0 and C24 genome assemblies [27] using the lastz programme with default parameters and the chaining (--chain) option. Best reciprocal hits (orthologues) were selected when (i) lastz alignments showed at least 90% reciprocal coverage with Col-0 genes, (ii) lastz alignments showed at least 95% identity, (iii) only one lastz best score per accession could be identified. Finally, we filtered out the candidates, which positions in contigs, were flanked by <500 bp upstream and downstream DNA. This resulted in the selection of 23,878 and 24,256 Col-0 orthologues in Bur-0 and C24, respectively. These were further filtered following expression data by selecting genes supported by at least three tilling array probes and other criteria (see ref. 32 , list of selected genes kindly provided by Dr Xi Wang). For each pair of orthologous genes, differences in expression levels were calculated using normalized tiling array data by subtracting the Col-0 expression level to the one of the orthologue from Bur-0 or C24 accession. How to cite this article: Maumus, F. and Quesneville, H. Ancestral repeats have shaped epigenome and genome composition for millions of years in Arabidopsis thaliana . Nat. Commun. 5:4104 doi: 10.1038/ncomms5104 (2014).